Nanophotonic control of circular dipole emission Controlling photon emission by single emitters with nanostructures is crucial for scalable on-chip information processing. Nowadays, nanoresonators can affect the lifetime of linear dipole emitters, while nanoantennas can steer the emission direction. Expanding this control to the emission of orbital angular momentum-changing transitions would enable a future coupling between solid state and photonic qubits. As these transitions are associated with circular dipoles, such control requires knowledge of the interaction of a complex dipole with optical eigenstates containing local helicity. We experimentally map the coupling of classical, circular dipoles to photonic modes in a photonic crystal waveguide. We show that, depending on the combination of the local helicity of the mode and the dipole helicity, circular dipoles can couple to left- or rightwards propagating modes with a near-unity directionality. The experimental maps are in excellent agreement with calculations. Our measurements, therefore, demonstrate the possibility of coupling the spin to photonic pathway. Control of the emission properties of circular dipole sources, where the phase of the orthogonal linear dipole components cannot be neglected, with a scalable nanophotonic interface would constitute a tremendous step towards viable, on-chip quantum information-processing. This control would allow for manipulation of the emission properties associated with the long-lived spin states of solid-state emitters, such as quantum dots [1] , [2] , [3] , [4] and nitrogen vacancy centres [5] , [6] , [7] , as their orbital angular momentum-changing decay to specific spin states is associated with the helicity of circular transition dipoles [8] , [9] ( Fig. 1a ). Furthermore, if nanophotonic structures could be interfaced with spin qubits, all the lessons learned from the study of how such structures interact with linear dipoles to, for example, control their decay rates [10] , [11] , [12] or the directionality of their emission [13] , [14] could be immediately applied. With such an interface one could couple, or even entangle, solid-state emitters to photonic pathways, essentially encoding the quantum information of a long-lived solid-state qubit on a versatile flying qubit [15] , [16] , allowing for a new avenue towards quantum information-processing elements. 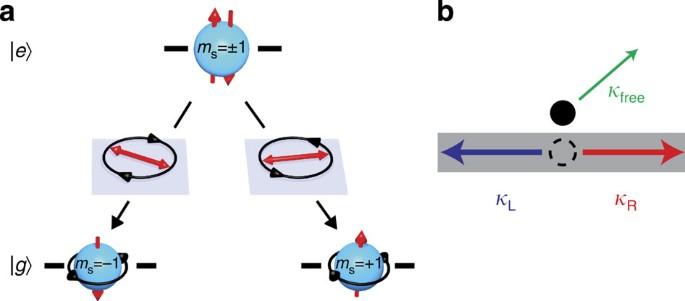Figure 1: Introductionary schematics. (a) Sketch of an emitter prepared in an excited state () that is a superposition ofms=−1,ms=+1, decaying with equal probability to either of the two opposite spin ground () states37. The transition between the two levels, a quantum process, results in the emission of a photon. This emission can be thought of as occurring because of a transition dipole (middle row), which arises because of the redistribution of charges in the emitter during the transition. This decay is associated with a circular transition dipole whose helicity is determined by the ground state to which the emitter decays, as sketched in the middle row, and the emission of a circularly polarized photon37. (b) A dipole placed inside (dashed circle, as is the case for QDs) or near (black dot, as is the case for our near-field probe) a PhCW can radiate into three channels (coloured arrows). These channels are labelled by L, R and free, with the corresponding ratesκL,κRandκfree, which indicate the emission efficiency into the left- and rightwards propagating modes and free space, respectively. Ifκi=1 where i=R, L, free, all photons are emitted into channel i. In our experiment we anticipate thatκfree>κR+κL. Importantly,κLandκRcan depend on dipole orientation and helicity, the directionality of the emission is (κL−κR)/(κL+κR). Figure 1: Introductionary schematics. ( a ) Sketch of an emitter prepared in an excited state ( ) that is a superposition of m s =−1, m s =+1, decaying with equal probability to either of the two opposite spin ground ( ) states [37] . The transition between the two levels, a quantum process, results in the emission of a photon. This emission can be thought of as occurring because of a transition dipole (middle row), which arises because of the redistribution of charges in the emitter during the transition. This decay is associated with a circular transition dipole whose helicity is determined by the ground state to which the emitter decays, as sketched in the middle row, and the emission of a circularly polarized photon [37] . ( b ) A dipole placed inside (dashed circle, as is the case for QDs) or near (black dot, as is the case for our near-field probe) a PhCW can radiate into three channels (coloured arrows). These channels are labelled by L, R and free, with the corresponding rates κ L , κ R and κ free , which indicate the emission efficiency into the left- and rightwards propagating modes and free space, respectively. If κ i =1 where i=R, L, free, all photons are emitted into channel i. In our experiment we anticipate that κ free > κ R + κ L . Importantly, κ L and κ R can depend on dipole orientation and helicity, the directionality of the emission is ( κ L − κ R )/( κ L + κ R ). Full size image Clearly, tremendous benefits can be obtained from a controlled interface of nanophotonics with spin states of emitters. Ideally, such an interface will be deterministic, meaning that all emissions are into the desired modes of the nanophotonic structure and not into free space ( Fig. 1b , κ free =0), and that each distinct spin state of the emitter is coupled to a single photonic pathway (either κ L =0 or κ R =0 depending on the emitter spin). The former requirement can be met by, for example, placing a quantum emitter inside a photonic crystal waveguide, which enables the extraction of over 98% of the quantum dot (QD) emission [17] . The latter requirement has, to date, not been demonstrated, although researchers have recently shown preferential emission of QDs situated at the crossing of two ridge waveguides [9] . It was shown that, depending on the helicity of its circular transition dipole, a QD preferentially emits into two of the four exit waveguides. For a deterministic interface of emitter spin to the photon pathway, detailed knowledge of the projection of a circular dipole on highly structured optical eigenstates of a nanophotonic structure, which contain local helicity [18] , is required. Such knowledge is the key if the emitter is to be correctly positioned. In practice, the fine details of the optical modes are highly dependent on the geometry of the nanostructure, and hence are sensitive to imperfections. Moreover, fabricating emitters in precise locations on nanophotonic structures is a complex and challenging procedure, which ultimately imposes additional constraints on the feasibility of a solid-state to flying-qubit interface. For example, the interaction of the nanophotonic structure and the emitter must be relatively constant over an area defined by the precision with which the emitter can be placed, typically on the order of tens of nanometres [19] , [20] . Consequently, a demonstration of a viable nanophotonic interface for solid state and flying qubits must fulfil two requirements. First, directional coupling between a circular dipole and a photon pathway must be observed on a nanophotonic structure. Second, a full spatial mapping of the interaction of the dipole and this structure must be created. Here we use a classical, tunable dipole source to demonstrate near-unity correlation of the combination of circular dipole helicity and the direction in which photons are emitted into a silicon photonic crystal waveguide (PhCW). First, we experimentally show that the radiation from the tip of a near-field optical microscope probe can mimic that of a linear transition dipole. Subsequently, we extend this method to emulate the emission of a circular transition dipole, that is, one that is associated with a change in an emitter’s spin state. By scanning this tunable source we create high-resolution spatial maps of its emission into the PhCW, for different helicity circular dipoles. We show that the helicity of the light emitted by such circular dipoles in combination with the unique local helicity of the photonic eigenstates of the PhCW leads to deterministic directional emission. Specifically, without detecting κ free , we find positions where the directionality of the emission, which actually goes into the PhCW, that is, the magnitude of ( κ L − κ R )/( κ L + κ R ) is near unity, with the actual direction depending on the dipole helicity. We underpin these experimental observations with a rigorous theoretical framework that describes the radiation of circular dipoles near a PhCW. Because the emission of a photon by a transition dipole and a classical dipole into a PhCW is identical in the weak coupling limit, our result points the way towards a future scalable spin-to-pathway coupling. Emission control with photonic crystal waveguides The way in which an emitter, and in particular a quantum emitter, radiates when placed near a nanophotonic structure is a subject of intense research [10] , [11] , [12] , [13] , [14] , [21] , [22] , [23] . The decay of a two-level system, an inherently quantum process, is associated with a transition dipole ( Fig. 1a ), which arises because of charge redistribution that occurs in the emitter during the transition. The radiation of the transition dipole is identical to that of a classical dipole, except that a transition dipole only exists for the duration of a single radiation event. When an emitter is placed near a nanophotonic structure the radiation probability of the transition dipole is altered by the number of photonic states into which it can emit. If the nanophotonic structure is a PhCW, and the emitter is located in the air above its surface, the factor by which emission is changed relative to free space is ( Supplementary Note 1 ). where e L,R are the electric (magnetic) fields of the normalized left- and right-propagating modes of the PhCW that interact with the dipoles of orientation , which can be electric ( ) or magnetic ( ) in nature, or both. Here, r is the emitter position, ω is the emission frequency, a is the PhCW lattice period, n g is the group index, and the subscripts L and R explicitly show that F can depend on the direction (in our case: left or right) in which light propagates in the PhCW. Lastly, we note that this expression assumes that all emission is into the photonic crystal waveguide modes [24] . The (transverse electric) TE-like photonic crystal waveguide modes are typically tightly confined and, as a result, also feature a field component along the propagation direction orthogonal to the in-plane transverse component. As a result of the periodic structuring of the PhCW, the relative magnitudes and phases of these components vary strongly within one unit cell to the extent that within one unit cell most, if not all, manifestations of the ( x , y )-polarization ellipse are present [18] . Owing to the structural symmetry of PhCWs, the left- and rightwards propagating modes are related via . From equation (1) it is clear that for perfectly directional emission into the PhCW we need and , or vice versa , for certain positions r 0 . For circular dipoles to maximally directionally emit into the PhCW, therefore, we require positions where the left- and rightwards propagating modes are circularly polarized, but with the opposite helicities. Modification of linear dipole emission Photonic crystal waveguides, by virtue of their highly structured near-field distributions that locally sample all in-plane vectorial field orientations [18] , seem ideally suited to couple emission to pathway. Moreover, PhCWs can also slow down light [25] , enhancing emission when n g is large (equation (1), Fig. 2a ). This enhancement can be observed in the calculated presented in Fig. 2b (see Methods), for linear and emitting at the wavelengths marked in the dispersion relation ( Fig. 2a ). Similar maps quantifying the interaction of the PhCW with magnetic dipoles can be created ( Supplementary Note 2 ). For , the maximum enhancement factor changes from 1.6 at 1,575 nm ( n g =15) to 9.8 at 1,592 nm ( n g =120). Furthermore, we observe that with increasing n g high enhanced emission factors become available away from y =0 (dashed blue line in Fig. 2b ). This is expected since the PhCW modes typically spread out as the light slows down [25] , [26] . Importantly, for all n g , the maps of the linear dipole emission modification factor (not shown) are identical to those of . Therefore, for a linear dipole the emission is not directional. 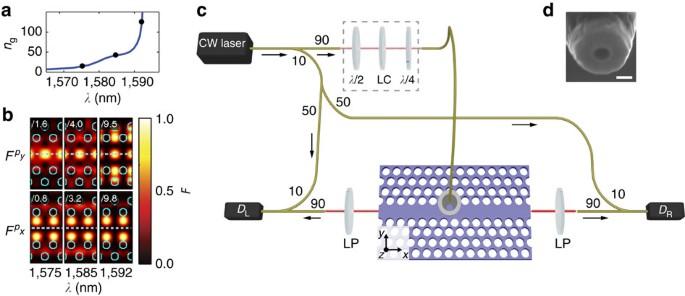Figure 2: Illumination-mode near-field microscope mimics dipolar emission. (a). Calculated group index of the PhCW. (b) Calculated enhanced emission factor (for light travelling to the left) forx-andy-oriented electric dipoles 20 nm above the PhCW, at wavelengths marked ina. Blue circles indicate the edges of the 110-nm holes in the PhCW and blue dashed lines indicate the centre of the waveguide. (c) Schematic of the near-field scanning optical microscope, operating in the illumination mode, that acts as a dipolar source. Light from a CW continuous-wave laser is split into reference and signal branches with the ratios shown. The polarization of the light in the signal branch, and hence the orientation of the dipole mimicked by the near-field scanning optical microscope probe, shown ind, is controlled by the polarization control scheme (dashed grey rectangle) that includes a half-wave plate (λ/2), a liquid crystal variable wave plate (LC) and a quarter-wave plate (λ/4). Light that couples to the PhCW travels to the left, or right, where it is detected inDLandDR, respectively, in an interferometric manner. (d) Scanning electron microscopy image of the near-field probe used in this work, with a 200-nm scale bar. Figure 2: Illumination-mode near-field microscope mimics dipolar emission. ( a ). Calculated group index of the PhCW. ( b ) Calculated enhanced emission factor (for light travelling to the left) for x- and y -oriented electric dipoles 20 nm above the PhCW, at wavelengths marked in a . Blue circles indicate the edges of the 110-nm holes in the PhCW and blue dashed lines indicate the centre of the waveguide. ( c ) Schematic of the near-field scanning optical microscope, operating in the illumination mode, that acts as a dipolar source. Light from a CW continuous-wave laser is split into reference and signal branches with the ratios shown. The polarization of the light in the signal branch, and hence the orientation of the dipole mimicked by the near-field scanning optical microscope probe, shown in d , is controlled by the polarization control scheme (dashed grey rectangle) that includes a half-wave plate ( λ /2), a liquid crystal variable wave plate (LC) and a quarter-wave plate ( λ /4). Light that couples to the PhCW travels to the left, or right, where it is detected in D L and D R , respectively, in an interferometric manner. ( d ) Scanning electron microscopy image of the near-field probe used in this work, with a 200-nm scale bar. Full size image We mimic the behaviour of a dipolar emitter using the emission from a 210-nm wide, near-field scanning optical microscope probe, which is known to act as a sort of continuous transition dipole [27] , [28] , [29] ( Fig. 2d ). We raster scan the probe in the sample plane at a height of 20 nm. While scanning, we collect the light coupled into the waveguide in a heterodyne detection scheme that gives us access to its phase ( Fig. 2c ). We use the phase information to Fourier-filter unwanted reflections from the waveguide end facets [18] , mapping out the excitation efficiencies of both the left- and rightwards propagating modes, and , respectively. Helicity-to-pathway coupling Because we wish to couple helicity to pathway, we need to confirm that we can control the orientation and phase of our dipole source. We start by showing that we can create any linear dipole ( λ free =1,575 nm), in this case by varying the orientation of our dipole from to . At this wavelength the PhCW interacts with magnetic dipoles in much the same way as it does with electric dipoles ( Supplementary Note 2 ). Consequently, we limit the following discussion to electric dipoles. We vary the orientation of the dipole by controlling the polarization of the light that we inject into our near-field probe, and show the measured and in Fig. 3a . These maps show that x - and y -oriented dipoles emit in drastically different ways into the PhCW, but as expected we do not observe directional emission. These measurements are in excellent agreement with the calculations ( Fig. 2b , and line cuts in Fig. 3a ). 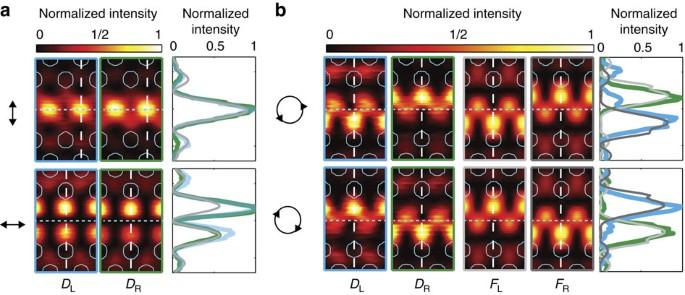Figure 3: Dipolar emission into a photonic crystal waveguide. (a) Experimentally collected emission maps collected with the left (DL, left column) and right (DR, right column) detectors, at 1,575 nm with linear dipoles (orientation indicated by the black arrows). Line traces are taken along the white dashed lines shown in the corresponding row, with the blue (green) lines corresponding to line traces throughDL(DR). Grey lines show cuts through the calculated(bottom panel) and(top panel), shown inFig. 2b. (b) Emission maps of right- (top row) and left-handed (bottom row) circularly polarized dipoles. In each row the two left (right) panels show experimental (theoretical) emission maps. As ina, the line traces (along the white dashed lines) correspond to cuts throughDL(DR), and are shown together with calculated cuts throughFL(dark grey lines) andFR(light grey lines). In all maps, light blue lines show the position of the holes of the PhCW and blue dashed lines mark the centre of the waveguide. Figure 3: Dipolar emission into a photonic crystal waveguide. ( a ) Experimentally collected emission maps collected with the left ( D L , left column) and right ( D R , right column) detectors, at 1,575 nm with linear dipoles (orientation indicated by the black arrows). Line traces are taken along the white dashed lines shown in the corresponding row, with the blue (green) lines corresponding to line traces through D L ( D R ). Grey lines show cuts through the calculated (bottom panel) and (top panel), shown in Fig. 2b . ( b ) Emission maps of right- (top row) and left-handed (bottom row) circularly polarized dipoles. In each row the two left (right) panels show experimental (theoretical) emission maps. As in a , the line traces (along the white dashed lines) correspond to cuts through D L ( D R ), and are shown together with calculated cuts through F L (dark grey lines) and F R (light grey lines). In all maps, light blue lines show the position of the holes of the PhCW and blue dashed lines mark the centre of the waveguide. Full size image To create circular dipoles, such as those associated with orbital angular momentum-changing transitions ( m s =±1 states, Fig. 1a ), we need to control the phase of our dipole source. Hence, we add a liquid crystal variable wave plate to our polarization control optics (LC in Fig. 2c , for details see Supplementary Note 4 ), which allows us to create sources. Strikingly, both the measured D L,R and the calculated F L,R for these circular sources ( Fig. 3b ) now exhibit a pronounced asymmetry. In fact, we observe that flipping either the emission direction ( D L or D R ) or dipole helicity [ or ] results in a mirroring of the excitation map about the middle of the waveguide ( y =0, dashed blue lines Fig. 3b ). For example, the emission of a right-handed dipole (top row of panels Fig. 3b ) is predominantly to the left when the dipole is placed over the bottom half of the waveguide ( y <0), and to the right when the dipole is located in the top half ( y >0). We take line cuts (along the dashed white lines in Fig. 3b ) to illustrate the strong relation between dipole helicity and the propagation direction of the photonic mode that it couples to. For both dipole handednesses, maximal emission in one direction corresponds to a minimum in the other. From both the calculations and the experiment we can determine the directionality of the coupling to the waveguide: ( κ L − κ R )/( κ L + κ R ). In both experiment and calculations we find positions of near-unity (0.98±0.02) directionality ( Supplementary Note 5 ). At these positions all emissions that are actually coupled into the PhCW are in a single direction that depends on the combination of the helicity of the dipole and the local helicity of the photonic mode. To explore whether our approach for coupling dipole helicity to pathway is a viable route towards future on-chip quantum technology, not only the directionality needs to be maximized, that is, by maximizing ( κ L − κ R )/( κ L − κ R ), but also the amount of emission into the waveguide needs to be optimized for a given κ free . In other words, a high directionality is only useful when it occurs at positions where the emission into the photonic mode is large. Please note that in our proof-of-concept with an emitter ~20 nm above the waveguide, we expect that κ free > κ L + κ R . However, the mode profile at a 20-nm height closely resembles the profile in the centre of the slab. It has been shown that when linear dipoles are placed in the centre of the slab, nearly all emissions can be extracted via the waveguide [17] . As a result, even though only a fraction of the emitted light is coupled to the waveguide, our measurements above the surface can still be used to determine whether the ideal positions for a future spin-to-pathway interface (high directionality plus optimal coupling) exist and what their location is. Hence, we examine the possibility of simultaneously obtaining perfect directional emission and κ L or κ R or equal to max( κ LCP,RCP ) near the PhCW surface. Consequently, we define the directional coupling efficiency, where the second line shows how we can extract Δ( r , ω ) from our measurements. In this equation, the subscripts denote propagation direction (L, R) or handedness (LCP, RCP) and max( D RCP,LCP ) is the maximum intensity found in any of and . 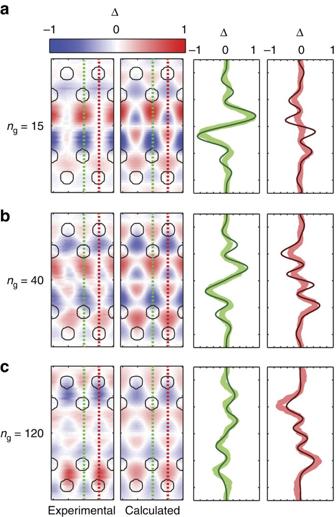Figure 4: Directional coupling efficiency. Experimental and calculated Δ maps for a combinedpandmdipole source at (a) 1,575 nm whereng=15, (b) 1,585 nm whereng=40 and (c) 1,592 nm whereng=120. Ina–c, experimental results are shown in the left panel, calculations in the middle panel and cuts along the dashed lines in the final panels. In these cuts, experimental (theoretical) data are shown in thick (thin) curves. Figure 4a (first panel) presents Δ( r , ω ) determined for emission at 1,575 nm, corresponding to the individually measured emission maps shown in Fig. 3b . Astonishingly, we observe relatively large regions where the helicity of the dipole almost perfectly determines the pathway that a photon will take, both to the left (Δ→1, red regions) and to the right (Δ→−1, blue regions). In fact, we observe a maximal directional coupling efficiency of , where the deviation from unity is largely because of experimental noise. Figure 4: Directional coupling efficiency. Experimental and calculated Δ maps for a combined p and m dipole source at ( a ) 1,575 nm where n g =15, ( b ) 1,585 nm where n g =40 and ( c ) 1,592 nm where n g =120. In a – c , experimental results are shown in the left panel, calculations in the middle panel and cuts along the dashed lines in the final panels. In these cuts, experimental (theoretical) data are shown in thick (thin) curves. Full size image We underpin our observations by calculating the theoretical directional coupling efficiencies, using equations (1) and (2) with . The calculations (second panel of Fig. 4a ) are in excellent agreement with the measurements, as can also be seen from the line cuts (right two panels) taken at positions of maximal directionality. The maximum theoretical directional coupling efficiency ( ) for this PhCW is 0.95, meaning that at this wavelength a circular dipole has the highest and most directional emission at the same locations (for a given κ free ). Because of the excellent agreement between experiment and theory, we can extend the calculations to the centre height of the PhCW slab. At the centre, where radiation to free space is almost completely suppressed [17] , we also predict near-unity directional coupling efficiency ( Supplementary Note 2 and 7 ). Finally, for completeness, we note that at this wavelength the calculated Δ for both electric and magnetic dipoles are almost identical ( Supplementary Fig. 6 ), with both peaking near unity. Tuning the directional coupling efficiency The optical properties of PhCWs can be tuned through geometry [30] . To explore this while using a single structure, we vary the excitation wavelength from 1,575 to 1,585 and 1,592 nm, where the calculated n g ’s are 40 and 120, respectively. For our PhCW, the modes, and hence F ( Fig. 2b ), at these wavelengths spread out away from the centre of the waveguide. Strikingly, in both the measurements and calculations at these higher n g ’s, regions of highly directional coupling appear away from the centre of the waveguide ( Fig. 4b ( n g =40) and Fig. 4c ( n g =120), Supplementary Note 5 ). Furthermore, as can be observed from the line cuts in Fig. 4 , as n g increases, the position of shifts from the central region of the waveguide to the area of the holes (and from the green to the red dashed line). Importantly, we observe that decreases as n g increases, from 0.8±0.1 at n g =15 to 0.6±0.1 at n g =40, and 0.7±0.1 at n g =102. This decrease in directional coupling efficiency is due to the combined emission of electric and magnetic dipoles that do not share identical Δ profiles ( Supplementary Note 3 and 5 ), and because, for the higher n g ’s, the maxima in directionality and emission amplitude are no longer located at the same position. It is, however, relatively simple to design a PhCW where over a broad range of n g ’s ( Supplementary Note 6 ). In conclusion, we have shown through classical measurements that a PhCW can be used to couple circular dipole helicity to emission direction, by exploiting the local helicity of the photonic modes. Experimentally, we observe a directionality of the coupling to the waveguide mode as large as 0.98±0.02. In other words, of the light from a circular dipole that is coupled to the waveguide the emission direction can be controlled through a combination of the helicity of the dipole and the local helicity of the mode. To assess the future potential of these points of maximal directionality, we also determine the directional coupling efficiency, which accounts for both the emission directionality and the amount of light coupled into the waveguide relative to the maximal coupling for a given coupling to free space. We experimentally find a directional coupling efficiency of 0.8±0.1, with a theoretical limit of unity, which can be found in a relatively large region. We demonstrate that this directionality is broadband, spanning 10’s of nms, and can be observed at a large range of n g ’s, even for a single PhCW. Furthermore, we demonstrate efficient directional coupling of both electric and magnetic emitters to the PhCW, making our results relevant for quantum emitters such as magnetic molecules [31] . The control over the emission direction of circular dipoles, as presented here, needs to be complemented by an efficient coupling to the nanophotonic structure ( κ free =0) in order to achieve a deterministic spin-to-pathway interface. Recent measurements have reported an almost perfect extraction of radiation from linear dipole sources (QDs) [17] , [32] , [33] . The local helicity of the photonic modes that we exploited above the surface is also present in the centre of the slab. Our concept should therefore be applicable to achieve the desired spin-to-pathway interface. Moreover, recent experiments have suggested that such an interface may be viable for systems other than QDs such as, for example, atoms [23] , [34] , [35] . Such an interface, be it for QDs, atoms or any other emitter, would allow for the entanglement of emitter spin to photonic pathway [16] , or could even be used to create quantum logic gates [15] , an important step towards future on-chip quantum optics applications. Fabricating the waveguide The fabrication of the photonic crystal waveguide begins with a silicon-on-insulator wafer (SOITEC, 200 nm Si layer/2 μm SiO 2 buffer). We have used electron-beam lithography to generate the required patterns in a resist (350 nm of ZEP 520-A, Zeon Chemicals). The patterns were transferred directly into the silicon layer of the wafer by reactive ion etching with an SF 6 /CHF 3 gas mix. After removing the remaining resist, the SiO 2 buffer was selectively removed from beneath the photonic crystal waveguide region with a dilute HF solution, thereby forming a silicon membrane in the area of the photonic crystal waveguide. The access waveguides that feed the photonic crystal waveguide are protected from the HF by a layer of S1818 (Shipley), which is spun on before the HF step. Calculation of the waveguide eigenmodes and dispersion The PhCW is a dispersion-engineered waveguide, where a missing row of holes in a 200-nm-thin silicon membrane perforated with a hexagonal pattern of holes (see Fig. 2c ). Light is confined in the plane of the waveguide by the photonic band gap of the surrounding holes, and is confined to the silicon slab by total internal reflection. Our waveguide has a lattice period a =420 nm and a hole radius of r =110 nm=0.262 a . The holes closest to the line defect are shifted outwards by 45 nm=0.11 a . The waveguide eigenmodes e L ( r , ω ) and eigenfrequencies are calculated with the freely available MIT Photonic Bands [36] , which determines the eigenmodes of the structure using a plane-wave basis set and periodic boundary conditions. We have used a supercell of dimensions , where h is the thickness of the Si slab, which is large enough to avoid interactions between neighbouring supercells. The calculations use a grid-size of a /16, which ensures convergence of the eigenvalues to better than 0.1%. We used a refractive index of Si of 3.48, suitable for wavelengths around 1,580 nm. How to cite this article: le Feber, B. et al. Nanophotonic control of circular dipole emission. Nat. Commun. 6:6695 doi: 10.1038/ncomms7695 (2015).